Sea surface temperature contributes to marine crocodylomorph evolution During the Mesozoic and Cenozoic, four distinct crocodylomorph lineages colonized the marine environment. They were conspicuously absent from high latitudes, which in the Mesozoic were occupied by warm-blooded ichthyosaurs and plesiosaurs. Despite a relatively well-constrained stratigraphic distribution, the varying diversities of marine crocodylomorphs are poorly understood, because their extinctions neither coincided with any major biological crises nor with the advent of potential competitors. Here we test the potential link between their evolutionary history in terms of taxic diversity and two abiotic factors, sea level variations and sea surface temperatures (SST). Excluding Metriorhynchoidea, which may have had a peculiar ecology, significant correlations obtained between generic diversity and estimated Tethyan SST suggest that water temperature was a driver of marine crocodylomorph diversity. Being most probably ectothermic reptiles, these lineages colonized the marine realm and diversified during warm periods, then declined or became extinct during cold intervals. Crocodylomorphs today show relatively narrow temperature tolerances, and their geographic distribution, whether on land or in the sea, is limited by temperature range. They are essentially tropical to subtropical organisms ( Alligator mississippiensis and Alligator sinensis being also known from warm-temperate zones) and their distribution in ancient environments is usually taken as an indication of tropical to subtropical temperatures [1] , [2] , [3] , a crucial adjunct to climate models for the Cretaceous and Cenozoic [4] . This assumption that crocodylomorphs are always indicators of tropical to subtropical conditions is based on their present distribution. Indeed, crocodylomorphs are unique among Mesozoic marine reptiles because some of them have living relatives. However, in the past, crocodylomorphs showed a far wider range of habitats and adaptations than seen among their modern counterparts. Most marine reptiles of the Mesozoic have no modern analogues, and processes affecting their rise and demise have been much debated in the context of covariation of palaeodiversity and sampling proxies [5] , [6] , [7] . The bias hypothesis (that is, errors induced by human collection or geological preservation) was put forward as the main explanation for palaeodiversity variation in Mesozoic marine reptiles [5] . Closer analysis suggested differences in the fossil records of the shelf and deep ocean, and that shallow marine tetrapod diversity was better explained by the extent of flooded continental areas than by sampling error [6] . More recently, it has been proposed that the extended extinction of unrelated marine reptile clades over the early Cretaceous could equally be explained by climatic or biotic factors exclusive to a given clade [7] . Another possibility is that marine reptile diversity could indirectly result from global changes in ocean chemistry, deeply scrambling the biomass and the structure of trophic chains, thus impacting again the diversity at the top of the food chain. There is therefore no clear consensus about the role of extrinsic versus intrinsic factors on marine reptile palaeodiversity in the Mesozoic. To test the control of the two major factors, seawater temperature or sea-level variations, on the diversity of marine crocodylomorphs, we have established a diversity database ( Supplementary Data 1 ) of marine crocodylomorphs at the generic level using all published occurrences worldwide from the Early Jurassic to the Late Eocene and compared them with published sea-level curves and to an updated sea surface temperature (SST) curve established from the oxygen isotope composition of fish teeth. Our analyses recover significant support for the covariation of seawater temperatures and the generic diversity of marine crocodylomorphs, excluding metriorhynchoids. A possible interpretation of these findings is that the evolution of most marine crocodylomorphs depends on environmental temperatures due to their ectothermic physiology. On the other hand, the radiation of metriorhynchoids during cold SST intervals suggests a different ecological strategy for this lineage. Palaeodiversity The stratigraphic ranges of marine crocodylomorphs across the studied time interval do not overlap, with the exception of marine eusuchians and Dyrosauridae, both of which appeared at the very end of the Cretaceous. No marine crocodylomorph has ever been reported from two intervals of the Cretaceous, the Hauterivian–Albian and the Coniacian–Campanian. These gaps in the fossil record can be considered as true absences because marine deposits of these ages are abundant (Paleobiology Database (PaleoDB) data) and have yielded remains of other marine reptiles, including ichthyosaurs, plesiosaurs or mosasaurs [5] , but have never yielded any crocodylomorphs. Thalattosuchians comprise the first marine radiation, with three genera recorded in the Toarcian, followed by a collapse in diversity during the Aalenian. This apparent peak is an artefact of preservation due to a typical Lagerstätte effect [5] , further expressed with the absence of record in the Aalenian, only recently recognized from new discoveries of other marine vertebrates [8] , [9] . A crocodylomorph assemblage containing both metriorhynchoids and teleosaurids existed at least since the Bajocian when the first alleged metriorhynchoids are recorded. From then, thalattosuchian diversity peaked in the Callovian with seven genera. A diversity drop is recorded between the Callovian and the Oxfordian. The metriorhynchoid burst in diversification took place during the Kimmeridgian–Tithonian interval, with five and seven genera recorded respectively. Although metriorhynchoids flourished, the diversity of teleosaurids for this same interval dwindled to only two genera, Machimosaurus and Steneosaurus . No teleosaurid has been reported thereafter. Finally, metriorhynchoid diversity dropped in the Berriasian with two genera and the clade disappeared during the early Hauterivian [10] , [11] , [12] . Thalattosuchians have never been reported from younger rocks. The present data compilation shows a gap in the record of marine crocodylomorphs from the early Hauterivian to the Cenomanian, when some pholidosaurids colonized the marine environment in the Cenomanian. They are not recorded after the Coniacian. The last radiation of crocodylomorphs into the marine environment is Maastrichtian in age, with five genera of Dyrosauridae and two genera of gavialoid eusuchians. Both Dyrosauridae and gavialoids survived the end-Cretaceous events, Dyrosauridae becoming extinct some time during the Ypresian. On the other hand, eusuchians seem to have radiated successively again during the Eocene, Oligocene and Miocene, as gavialoids. Tests of correlation In comparisons of different data treatments, Spearman rank correlation tests suggest some correlation of the palaeodiversity signal with the explanatory time series. 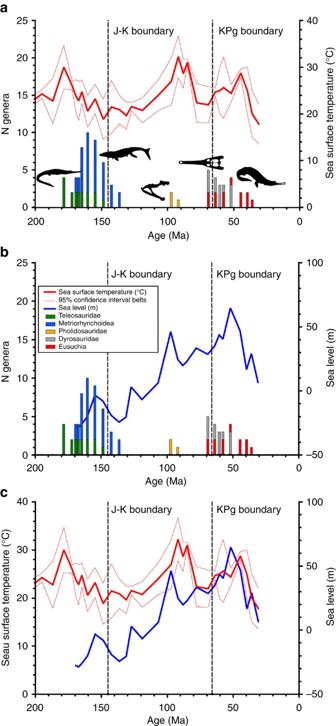Figure 1: Phylogenetically corrected generic diversity counts of marine crocodylomorphs. SST curve (a) and sea-level curve of Milleret al.13(b) plotted against geological time. SST and sea-level curve of Milleret al.13are compared (c), showing a close but imperfect co-variation. Out of the five explanatory time series, SST shows the greatest number (7) of significant results for the correlation tests against the response variables ( Table 1 ). This is closely followed by the data for sea-level reconstruction by Miller et al . [13] , with five significant results. Then, the sea level estimate of Haq et al . [14] shows only one significant correlation with the response variable. Finally, the two subsequent explanatory variables (PaleoDB marine formations and COSUNA (Correlation of Stratigraphic Units of North America) formations) show nonsignificant correlations with the response variables. Table 1 Correlations of potential explanatory variables with different metrics representing marine crocodylomorph diversity through the Mesozoic and Paleogene. Full size table There appears to be no good match when either raw crocodylomorph species diversity counts or phylogenetically corrected generic diversity counts are compared with SST. The tested relations remain unmatched when applying various data transformations (time-scaling, logarithmic and generalized differencing). Significant correlations between SST and the response variables appear when metriorhynchoid crocodylomorphs are excluded from the diversity count (no metriorhynchoids (NM) data set). In terms of strength of correlation, Log 10 (NMcroc) offers the best result, which is as good as the correlation coefficients recovered for the sea-level estimate of the Miller et al . [13] curve versus the response variables. Nevertheless, SST stands out from the sea-level estimate of Miller et al . [14] when the response variables are phylogenetically corrected, with four significant correlation coefficients (>0.36) explained by SST versus one significant correlation coefficient (0.405) for Miller sea level ( Table 1 ). Noteworthy in the results are significant positive correlation coefficients obtained when considering SST or the sea-level estimate of Miller et al . [13] against generalized differences of the diversity data set without metriorhynchoids (generalized difference (GD) NMcroc and phylogenetically corrected diversity (GD) NMcroc in Table 1 ). After correction for multiple comparisons with the Benjamini–Hochberg and Bonferroni corrections, we found that all significant correlations ( Table 1 ) ceased to be significant. Perhaps the corrections were too harsh, or at least any correlations that exist between the marine crocodylomorph fossil record and the putative physical drivers are weak. There are clearly problems with the time bins and palaeodiversity sample sizes used here. The temporal distribution of the fossil record of marine crocodylomorphs is not as resolved as that of the SST data. This means that variations in temperatures within these time bins cannot be compared with the evolution of diversity at a finer stratigraphic scale, simply because the stratigraphic distribution of the marine vertebrates can only be inferred using ghost ranges. Nevertheless, these results do not invalidate the simple observation that marine crocodylomorphs are present in the marine environment when warm SST prevail, but are absent when cold SST are recorded. These findings are discussed below. No significant correlation between marine crocodylomorph diversity and PaleoDB marine formations is observed, under any manipulation of the time series, therefore suggesting that the ups and downs in marine crocodylomorph diversity are not dominated by geological sampling, but indicate some aspects of the original diversity signal and ought to be explained by other external factors. The absence of significant correlation between marine crocodylomorph diversity and the metric for continental flooding (COSUNA) contrasts with previously published results, although it should be noted that the present diversity data sets are necessarily small. A strong negative correlation was found between non-flooded surface area and the taxic diversity of shallow environments [6] , a result predicted by the inverse relation between non-flooded surface area and the number of shallow marine habitats. As predicted by these results [6] , a positive and significant correlation would be expected in our results between COSUNA and marine crocodylomorph diversity, but this is not the case. Our data set focuses on one group, marine crocodylomorphs, versus all marine reptiles, as in the case of Benson and Butler [6] , who lump marine crocodylomorphs among shallow marine tetrapods. Broad feeding scope and enhanced mobility in marine crocodylomorphs are strong indications that their diversity should not have been significantly influenced by habitat modification, despite significant modifications of the palaeogeography during the time under investigation. Moreover, because of their freshwater origin, marine crocodylomorphs were certainly able to live in freshwater drainages, as identified in some cases [15] , and could use the various food resources available in the freshwater habitat. The combined role of ecology, physiology or behaviour may therefore explain why marine crocodylomorph diversity does not show good correlation with continental flooding. Pierce et al . [16] suggested that thalattosuchian extinction in the Early Cretaceous was driven by sea-level fall. The present results show that marine crocodylomorph diversity is at least partly affected by sea-level variations. It is indeed expected that coastal palaeogeography can be significantly modified by sea-level changes, resulting in the appearance of new habitats and marine barriers, differing in size and marine connection through time (for example, ref. 17 ). How this affected crocodylomorph diversity is unknown but should be considered. Correlations computed on the total diversity data set of marine crocodylomorphs with the sea-level estimates are not significant. On the other hand, exclusion of metriorhynchoids from the data set leads to five significant correlations with the sea-level estimates of Miller et al . [12] and a single significant correlation with the sea-level estimates of Haq et al . [14] These results underline that marine crocodylomorphs with varying adaptations for offshore (for example, teleosaurids) or pelagic swimming (metriorhynchoids) may be affected differently by sea-level variation. For instance, metriorhynchoid diversity alone seems to be affected by sea-level variation of Miller et al . [12] ( Fig. 1b ), but there is no correlation (Spearman’s ρ =0.577, P =0.13), and perhaps the narrow temporal range (Pliensbachian–Valanginian) prevents meaningful statistical testing. However, this hypothesis is unequally supported by the two available sea-level data sets (the one from Miller et al . [13] being incomplete from the Hettangian to Aalenian) and loses much support when the data set is phylogenetically corrected ( Table 1 ). Although sea-level variation might partly explain the diversity of marine crocodylomorphs, it is noteworthy that sea level is both influenced by global tectonic activity (tectonoeustasy) and the growth and decay of polar ice caps (glacioeustasy). As the extension of the polar ice is ultimately controlled by global climate, a drop in sea level could be related indirectly to a drop in marine crocodylomorph diversity, but the underlying cause would be temperature change ( Fig. 1c ). Figure 1: Phylogenetically corrected generic diversity counts of marine crocodylomorphs. SST curve ( a ) and sea-level curve of Miller et al . [13] ( b ) plotted against geological time. SST and sea-level curve of Miller et al . [13] are compared ( c ), showing a close but imperfect co-variation. Full size image Although based on now obsolete diversity counts, strong evidence for the influence of climate on the evolution of crocodylomorphs has previously been detected [4] . It is expected that crocodylomorphs, as ectotherms, are affected by temperature changes; this is reflected in the marine environment by the temperature of their living medium (SST). No correlation between SST and total marine crocodylomorph diversity is observed ( Table 1 ), a result drastically different when metriorhynchoids are excluded from the data set ( Table 1 ). In this case, significant correlations are observed both with and without phylogenetic correction. The average significant correlation value for SST is 0.380. Such a value implies that SST can only partially explain the diversity of some marine crocodylomorphs and suggests that with the exclusion of metriorhynchoids, they were only able to colonize the marine environment when ambient temperatures were favourable. According to the present knowledge of the fossil record, the marine environment was left vacant twice for several million years by crocodylomorphs, in the Hauterivian–Albian and Coniacian–early Campanian intervals. Possibly, the marine environment was not habitable. It is notable that crocodylomorphs colonized the marine environment at the beginning of warming phases, with Thalattosuchia in the Toarcian, Pholidosauridae in the Cenomanian and Eusuchia, and Dyrosauridae in the Maastrichtian. On the other hand, some drops in crocodylomorph diversity correspond to temperature declines such as that of the Callovian affecting thalattosuchian diversity or the Valanginian–Hauterivian boundary affecting metriorhynchoids. Concerning the extinction of Pholidosauridae in the Turonian and Dyrosauridae in the Ypresian, a clear match between SST and diversity is absent, even when considering fine-scale SST variations reconstructed using other proxies [18] , [19] . Among the considered marine crocodylomorph lineages, the metriorhynchoids clearly stand out with an explosive radiation at the end of the Jurassic, when SSTs continued to decrease. Comparatively, the other thalattosuchian group, the teleosaurids, did not radiate and even went extinct before the Berriasian. Metriorhynchoids appear to be morphologically different from any other marine crocodylomorphs, thus inviting discussion about physiological adaptations in these different lineages (see below). The statistical assessments retrieved in this study did not yield 1:1 correlations between SST and marine crocodylomorph diversity, and as discussed below other factors might be involved in the fluctuations in marine diversity. The aim of this study is not to prove that SST could solely account for evolutionary patterns in climate-sensitive lineages, but rather to stress the existence of a window of optimal temperatures in which these marine animals could thrive, as defended in earlier studies [4] . SST can be interpreted as a limiting factor, allowing crocodylomorphs to colonize new environments when temperatures become favourable; or preventing crocodylomorphs from widely thriving when temperatures fall. It is noteworthy that increasing marine water temperatures also boost both biomass and biodiversity, thus increasing the amount of resources for marine crocodylomorphs. Within that frame, other factors, including biotic ones could impede speciation. One factor coming to mind is competition for resources or territory among predators [20] . Illustrating this, the demise of Pholidosauridae, and then of Dyrosauridae might be paralleled with the rise of other large marine predators: mosasaurs in the mid-Cretaceous or archaeocete marine mammals in the Paleogene. However, explaining the turnover of vertebrates by competition for resources or territory should take into account the body size factor. Body size is responsible for niche partitioning in large predators [21] and it is unlikely that pholidosaurids or dyrosaurids might have been worried by the small size of the first mosasaurs and the first archaeocetes. Moreover, there are numerous instances of marine crocodylomorphs coexisting with other large marine reptiles [7] , [9] . Therefore, invoking competition for resources or territory appears unlikely as an explanation for the demise of marine crocodylomorphs. Physiological specificities could represent other factors explaining the diversity pattern of marine crocodylomorphs. The prediction that ancient marine crocodylomorphs were sensitive to seawater temperature variation is partly but not entirely recovered in our results. The fact that ancient marine crocodylomorphs were, as extant ones, ectotherms would require a full match between SST evolution and patterns of radiation–extinction of the different crocodylomorph groups. Of particular relevance to the recovered mismatch are Metriorhynchoidea, whose diversity does not match SST evolution. Indeed, the Metriorhynchoidea appeared to radiate in the pelagic environment when Teleosauridae died out and SST dropped at the end of the Jurassic. Whether metriorhynchoids retained ectothermic characteristics is questionable and unanswered, but could equally be linked to drastic physiological changes such as reproductive strategies. Metriorhynchoidea display extreme adaptations to marine life, with hypocercal tails and paddle-like limbs [22] , the latter clearly not suited for land crawling. Extant crocodylomorphs need to come back onto land to lay eggs, but if this could not be achieved by metriorhynchoids, a whole suite of physiological adaptations would have been required, including live birth. As speculative as it may be, this could explain their explosive radiation after the Callovian–Oxfordian temperature drop and their survival after the end-Jurassic, while Teleosauridae drastically declined in diversity and then disappeared. Live birth was widespread among ichthyosaurs [23] and has only recently been reported for plesiosaurs [24] and mosasaurs [25] . In the first two groups, δ 18 O values of bone phosphate tissue support the hypothesis of body-temperature regulation [26] . Whether metriorhynchoids had some sort of endothermic capability would be consistent with our results, also supported by their inferred hypercarnivorous diet [27] , fulfilling the high metabolic demand for protein. Although this remains to be tested (for example, by analysing the δ 18 O composition of metriorhynchoid bone phosphate), an intermediate metabolism could explain both the delayed reaction to SST drops when teleosaurids disappeared, and also their demise at the Hauterivian–Valanginian boundary when SST may have dropped below metriorhynchoid tolerance. The temperature tolerance of metriorhynchoids would have been better suited for cold temperatures than that of other marine crocodylomorphs, but remained unparalleled to that of plesiosaurs and ichthyosaurs living in high-latitude cold environments [28] , [29] , [30] . No marine crocodylomorphs have ever been reported in these high-latitude marine environments of the Jurassic and Cretaceous, whereas they were abundant in contemporaneous lower latitude assemblages. This provides support for the first assumption that marine crocodylomorphs were ectotherms, and therefore their capacity to diversify in the marine environment was ultimately constrained by the evolution of SSTs. Diversity counts Marine crocodylomorph diversity counts were assessed at species and genus level. Occurrences extend over the Hettangian to the Rupelian ( Supplementary Data 1 ). To begin with, species counts were retrieved from the literature for the Dyrosauridae and the Eusuchia, and updated from Benson et al . [5] for the Thalattosuchia and Pholidosauridae. The species raw count was included in the statistical analysis and a second set of analyses excluded metriorhynchoids from the species count. To reduce taxonomic bias as much as possible, another set of data considered only genera. This is because across the different lineages of marine crocodylomorphs considered here, two have recently been revised in depth leading to a burst of previously overlooked species diversity [31] . Species diversity, and to a lesser extent generic diversity, are unbalanced when comparing recently revised groups such as metriorhynchoids or dyrosaurids, versus other groups such as the Teleosauridae, whose taxonomic content has not been revised recently [32] , [33] . Therefore, considering only genera in the data set allows us to smooth out diversity counts across different lineages. An additional approach was applied to this generic data set for further refinement of the diversity: phylogenetic correction, superimposed on the stratigraphy by filling ghost ranges of genera ( Supplementary Data 1 ). Phylogenetic corrections follow the topology recovered for Thalattosuchia [31] and the topology recovered for Dyrosauridae [34] . Pholidosauridae (two marine genera) are, in comparison with Thalattosuchia and Dyrosauridae, a relatively small marine radiation with a larger ancestral freshwater stock. For this reason, no phylogenetic correction could be applied here and only their ghost occurrence was added to the stratigraphic series. Finally, phylogenetic correction was not applied to marine Eusuchia due to their controversial phylogenetic relationships at the heart of the Gavialis / Tomistoma debate [35] . Therefore, only ghost ranges were added according to the stratigraphic distribution of taxa. Poorly known taxa from marginal setting A number of problematic crocodylomorphs were not included in the marine crocodylomorph diversity count because of uncertain taxonomic identity and limited occurrence at a single locality in a marginal marine setting. These taxa are: Aigialosuchus villandensis Persson [36] from the early Campanian of Blaksudden Ivö, which is fragmentary and may well have been washed out in marginal marine deposits together with dinosaurian teeth found in the same deposits. Moreover, according to the morphology described by Persson [36] , Aigialosuchus villandensis can be considered similar to contemporaneous freshwater eusuchians. Crocodileimus robustus Jourdan [37] from the Kimmeridgian of Cerin, France, possibly belongs to the Pholidosauridae but this has not been substantiated yet. Crocodileimus robustus occurs in a lagoonal mudstone and the presence of atoposaurids in the same locality points to episodes of continental washout into this environment. Although Pholidosauridae diversified during the early Cretaceous, they were restricted to freshwater environments. The genus Anglosuchus from the Great Oolite (Bathonian) of Peterborough, UK, has previously been referred to the Pholidosauridae [38] , [39] , [40] but these referrals have never been substantiated. The youngest teleosaurid was recorded from the Valanginian of southern France [41] . This specimen has recently been revised [42] and now referred to a metriorhynchid. The youngest record of Teleosauridae is therefore Tithonian in age, no record being substantiated for this group in the Cretaceous. Seawater temperature curve establishment SST curve for the Hettangian–Rupelian interval has been established using both published [26] , [43] , [44] , [45] , [46] , [47] , [48] , [49] , [50] , [51] and new oxygen isotope composition of fish teeth recovered from European, American, North African and Middle East localities corresponding to the Western Tethys realm ( Supplementary Data 1 ). To be comparable, δ 18 O p values were all normalized to the most recently accepted value of 21.7‰ for the international standard NBS 120c [52] . Values with maximum resolution at the substage level were selected and an average value for the whole stage was calculated. Seawater temperatures were then computed using the phosphate-water temperature scale [52] assuming an average δ 18 O value of the ocean of −1‰: Statistical assessment This data set is then compared with the SST curve ( Fig. 1a ) based on the compilation of new and published δ 18 O values of fish tooth apatite phosphate recovered from low to mid-latitude localities, and to sea level ( Fig. 1b ), which was recalculated for each stratigraphic interval defined in Gradstein et al . [53] along with the values obtained from Haq et al . [14] (Hettangian–Rupelian) and Miller et al . [13] (Bajocian–Rupelian). Marine crocodylomorph diversity is also confronted with another physical factor, which is a metric for continental flooding [5] compiled from MACROSTRAT (COSUNA [54] ). Finally, to test possible taphonomic bias in the diversity of marine crocodylomorphs, the number of marine geological formations was compiled from the PaleoDB and compared with the diversity data set. The stratigraphic framework of Gradstein et al . [53] is adopted here. We carried out a series of correlation tests to determine the relationship between marine crocodylomorph diversity and paleoclimate. We considered four forms of the diversity data, and for each of those, four variants on the data. The time series of crocodylomorph diversity was presented in these four formats: (1) total species diversity; (2) phylogenetically corrected generic diversity, including ghost ranges; (3) total species diversity minus metriorhynchoids; and (4) phylogenetically corrected generic diversity minus metriorhynchoids. Phylogenetic correction is commonly done for studies of fossil vertebrates [6] , [55] : this consists of plotting a cladogram against geological time, and adding Lazarus taxa (genera with a range above and below a time bin of interest) and ghost ranges (minimal implied range at the base of a lineage implied by older fossils in the immediate sister group). Each of the four data formats was further considered in four forms: (1) raw data; (2) time-corrected (total figures divided by durations of time bins); (3) logarithm (total data); and (4) generalized-difference (GD) total data. These modifications were to allow all possible corrections for variable time bin duration, for any large-scale deviations from the mean (logarithm transformation) and to distinguish overall trend from bin-by-bin variations (generalized-differencing). Pairwise tests of correlation were carried out between the response variables (diversity time series) and the various possible explanatory time series (the new SST data, the Miller sea-level curve, the Haq sea level curve, PaleoDB marine formation counts and COSUNA marine formation counts). Pearson, Spearman and Kendall correlation coefficients and significances were calculated using R software v.2.14.1 (R Development Core Team, 2011), as in earlier studies [56] . Further, we recorded raw significance values as well as those corrected for type II statistical errors, using the false discovery rate approach [57] , using an R script given in Benton et al . [51] , which runs numerous correlation tests with unadjusted and adjusted P -values. How to cite this article: Martin, J. E. et al . Sea-surface temperature contributes to marine crocodylomorph evolution. Nat. Commun. 5:4658 doi: 10.1038/ncomms5658 (2014).